The interaction between OsMADS57 and OsTB1 modulates rice tillering viaDWARF14 Rice tillering is a multigenic trait that influences grain yield, but its regulation molecular module is poorly understood. Here we report that OsMADS57 interacts with OsTB1 (TEOSINTE BRANCHED1) and targets D14 ( Dwarf14 ) to control the outgrowth of axillary buds in rice. An activation-tagged mutant osmads57-1 and OsMADS57 -overexpression lines showed increased tillers, whereas OsMADS57 antisense lines had fewer tillers. OsMIR444a- overexpressing lines exhibited suppressed OsMADS57 expression and tillering. Furthermore, osmads57-1 was insensitive to strigolactone treatment to inhibit axillary bud outgrowth, and OsMADS57 ’s function in tillering was dependent on D14 . D14 expression was downregulated in osmads57-1 , but upregulated in antisense and OsMIR444a- overexpressing lines. OsMADS57 bound to the CArG motif [C(A/T)TTAAAAAG] in the promoter and directly suppressed D14 expression. Interaction of OsMADS57 with OsTB1 reduced OsMADS57 inhibition of D14 transcription. Therefore, OsMIR444a -regulated OsMADS57 , together with OsTB1 , target D14 to control tillering. This regulation mechanism could have important application in rice molecular breeding programs focused on high grain yield. Transcription factors of the MADS-domain family (named for yeast MCM1, plant AGAMOUS and DEFICIENS, and mammal Serum Response Factor) are highly conserved among fungi, animals and plants. Genetic interactions of MADS-box family members are involved in flowering, floral organ identity and development, embryogenesis and meristem differentiation. In rice, the genetic interactions among the four AG subfamily members, OsMADS3 , OsMADS13 , OsMADS21 and OsMADS58 , determine the identity of floral organs [1] . OsMADS6 interacts with SUPERWOMAN1 , OsMADS3, OsMADS58 , OsMADS13 and DROOPING LEAF to control floral organ identities and meristem fates [2] . At the protein level, MADS proteins generally interact with themselves or other proteins to form homodimer or heterodimer for performing their functions [3] , [4] , [5] . MADS-domain proteins recognize and bind to specific palindromic DNA sequences with a CArG core consensus element to regulate the expression of target genes [4] , [6] , [7] , [8] . The ‘floral quartet model’ suggests that floral organ identity regulators of the MADS-box family assemble into organ-specific quaternary transcription factor complexes to control the identity and development of floral organs. However, less is known about how the transcription factors and their targets function in planta . With regard to spatial expression patterns of MADS genes, it is worth noting that several genes in the MIKC c -type group (MEF-like (M-), intervening (I-), Keratin-like (K-) and C-terminal (C-) domains), the AGL12 -like clade, the STMADS11 -like clade and the AGL17 -like clade are predominantly expressed in vegetative tissues. In rice, AGL17 -like clade genes, including OsMADS23 , OsMADS25 , OsMADS27 , OsMADS61 and OsMADS57 ( [9] ) exhibit this pattern and are expressed predominantly in vegetative tissues. This implies a unique function in vegetative development [9] , [10] . However, the specific mechanism of MADS protein interaction with target genes for the induction of function in vegetative organ development is poorly understood. MADS and TCP ( T EOSINTE BRANCHED1 ( TB1 ) from maize, C YCLOIDEA from Antirrhinum and P ROLIFERATING CELL FACTOR from rice) have been shown to cofunction in determining meristem identity and control organ morphogenesis [11] . In floral organogenesis, MADS genes primarily mediate organ identity, while TCP genes regulate floral meristem symmetry. TCP genes also participated in the regulation of vegetative branching patterns [12] , [13] , [14] . TB1 was under strong selection as maize became an agricultural cultivar, and has been shown to function as a reducer of axillary bud growth in maize, rice and Arabidopsis [12] , [13] , [15] . The expression of AGL17 -like clade genes in vegetative tissues hints that they may also have a role in the differentiation of axillary buds. However, there is currently no evidence to support this supposition, and it remains unclear how TCP and MADS coordinate the regulation of branching in plants. Tillering or branching genes function during the initiation of morphogenesis and/or the outgrowth of axillary buds. A series of shoot-branching mutants have been identified in diverse plant species, including max ( more axillary growth ) in Arabidopsis, rms ( ramosous ) in pea, dad ( decreased apical dominance ) in petunia, tb1 in maize and dwarf ( d ) in rice [12] , [15] , [16] , [17] , [18] , [19] , [20] . The rice mutant moc1 ( monoculm 1 ) has characteristic monoculms, lacking any tillers. The transcription factor MOC1, together with MIP1, controls the initiation and outgrowth of axillary buds in rice [21] . Degradation of MOC1 with APC/C TAD1/TE in a cell-cycle-dependent manner mediates rice tillering [22] , [23] . In contrast to these genes that reduce tillering, there are a series of rice mutants that confer an increased number of tillers. These include d3 , d10 , d17 , d33 , ostb1 , d27 and d14 , and their corresponding genes are suggested to be involved in the regulation of axillary bud outgrowth for tillering in rice. D14 functions in strigolactone (SL) signalling to control tillering, while D27 functions in SL biosynthesis [19] , [24] , [25] . Several components of the SL biosynthesis pathway, including carotenoid cleavage dioxygenase (CCD)7, CCD8, MORE AXILLARY GROWTH1 (MAX1) and D27, have been implicated in axillary bud outgrowth [16] , [17] , [18] , [19] , [26] , [27] . Expression of D27 is directly regulated by GRAS transcription factors, NODULATION SIGNALLING PATHWAY1 (NSP1) and NSP2 in Medicago truncatula and rice [28] . Genetic and biochemical studies suggest that D14/D88/HTD2 functions in SL biosynthesis or signal transduction, and that MAX2/D3/RMS4 and DAD2/D14 perceive and transduce the signals [20] , [24] , [25] . However, it remains unclear how such genes are directly coordinated to function in axillary bud outgrowth in plants. Here we explore the role of OsMADS57 in the regulation of tillering using transgenic lines and related mutants. Our results show that OsMADS57 is negatively regulated by miR444a, and that OsMADS57 subsequently negatively regulates the expression of D14 , thereby affecting tillering. This negative regulation by OsMADS57 is suppressed by interaction with OsTB1, leading to the balanced expression of D14 for tillering. The osmads57-1 mutant has increased tillering OsMADS57 was predicted to encode a protein containing a MADS-box domain, a variable I region, a conserved K-box domain and a C-terminal region ( Fig. 1a ). Phylogenetic analysis grouped OsMADS57 into the AGL17 -like lineage ( Fig. 1c ) that is predominantly expressed in vegetative tissues [9] , [29] . The T-DNA insertion mutant line PFG_3A-05432.L, named henceforth as osmads57-1 , was obtained from RiceGE, the Rice Functional Genomics Express Database of Korea [30] . The T-DNA was inserted into P0617A09 at the 86,816-bp position in the rice genome, where the predicted gene OsMADS57 is annotated. DNA gel blot analysis showed one copy of the T-DNA in the genome ( Supplementary Fig. S1b ). The gene contains eight exons and seven introns and is 6,094 bp in total length ( Fig. 1b ). The T-DNA insertion position is 5,275 bp from the transcriptional initiation site in OsMADS57 ( Fig. 1b and Supplementary Fig. S1a ). 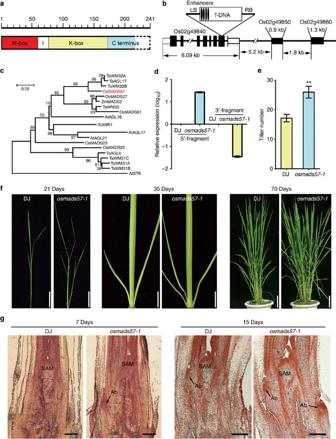Figure 1:OsMADS57structure and phenotype of theosmads57-1. (a) OsMADS57 sketch; MEF-like (M-box); intervening (I); Keratin-like (K-box); Carbon (C)-terminus domains; Dashes-box, the truncated-part; Scale numbers, amino-acid residues. (b) T-DNA insertion inOsMADS57(Os02g49480). (c) Phylogenetic tree ofAGAMOUS-like17genes. (d) Transcript patterns inosmads57-1at 15 DAG. (e) Tiller numbers at 70 DAG. Values represent means±s.e. of ten plants. **P<0.01 by Student’st-test. (f) Tillering phenotypes in various stages. Scale bar, 5 cm. (g) Longitudinal sections of shoot meristems (SAM) and axillary buds (Ab). Scale bars, 100 μm. Figure 1: OsMADS57 structure and phenotype of the osmads57-1 . ( a ) OsMADS57 sketch; MEF-like (M-box); intervening (I); Keratin-like (K-box); Carbon (C)-terminus domains; Dashes-box, the truncated-part; Scale numbers, amino-acid residues. ( b ) T-DNA insertion in OsMADS57 (Os02g49480). ( c ) Phylogenetic tree of AGAMOUS -like 17 genes. ( d ) Transcript patterns in osmads57-1 at 15 DAG. ( e ) Tiller numbers at 70 DAG. Values represent means±s.e. of ten plants. ** P <0.01 by Student’s t- test. ( f ) Tillering phenotypes in various stages. Scale bar, 5 cm. ( g ) Longitudinal sections of shoot meristems (SAM) and axillary buds (Ab). Scale bars, 100 μm. Full size image The T-DNA insertion caused a fused open reading frame of 675 bp in osmads57-1 , rather than the original 726 bp open reading frame of OsMADS57 in wild type (WT; Fig. 1b and Supplementary Fig. S1c,d ). In the mutant, 24 amino-acid residues at the OsMADS57 C terminus were replaced with a peptide of 7 amino-acid residues encoded by the T-DNA to form a fusion protein, OsMADS57F ( Supplementary Fig. S1a ). OsMADS57F was predicted to contain the MADS-box domain, the I region and the K-box domain, but not the intact C terminus ( Fig. 1a ). The transcription level of a 5′-fragment of OsMADS57 was increased in the mutant, but a 3′-fragment was dramatically decreased ( Fig. 1d ). Therefore, osmads57-1 is a T-DNA insertion mutant that overexpresses the truncated OsMADS57. Unlike the other known MADS genes rice mutants, osmads57-1 did not have any significant alterations in floral organogenesis or development, except for crooked anthers and altered primary root growth compared with WT plants ( Supplementary Fig. S2 ). Primary root growth was repressed in the osmads57-1 mutant compared with WT plants until 7 days after germination (DAG; Supplementary Fig. S2a,b ). This significant difference disappeared after 14 days. The osmads57-1 mutant showed an obvious increase in the number of tillers from the 4th-leaf stage to the mature stage ( Fig. 1e ). Histological analysis revealed the appearance of outgrowth of axillary buds as early as 7 DAG in osmads57-1 , whereas this outgrowth was absent in WT Dongjin (DJ) ( Fig. 1g ). At day 15, osmads57-1 plants showed two axillary bud outgrowths, whereas WT showed only one. Therefore, enhanced expression of truncated OsMADS57 may cause accelerated emergence of axillary bud outgrowth in osmads57-1 plants. OsMADS57 and OsMIR444a are involved in axillary bud development To confirm the phenotypes further, we created six OsMADS57 -overexpression lines (OE) and three antisense transgenic lines (AS). Quantitative reverse transcription–PCR (qRT–PCR) assays revealed that OsMADS57 expression was enhanced in OE lines (for example, OE1) and suppressed in antisense lines (for example, AS3) compared with WT plants ( Fig. 2a ). Antisense line AS3 had fewer tillers than WT Zhonghua10 (ZH10). In contrast, the OE1 line had more tillers than ZH10 ( Fig. 2a ), without alteration in floral organogenesis ( Supplementary Fig. S2c ). Therefore, osmads57-1 is likely a gain-of-function mutant. 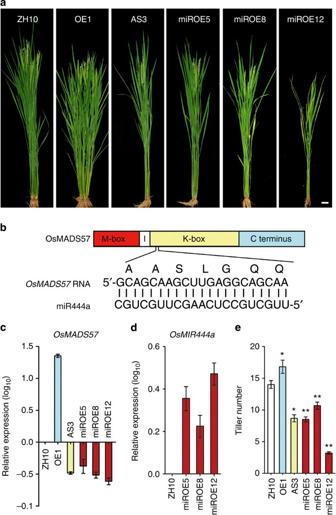Figure 2: Morphological comparison of the transgenic lines. (a) Tillering phenotypes. Scale bar, 5 cm. (b) miR444a and its target sequence sketch. (c,d) Relative expression in the transgenic lines. (e) Tiller numbers at 70 DAG. Values represent means±s.e. of ten plants. *P<0.05, **P<0.01 by Student’st-test. Figure 2: Morphological comparison of the transgenic lines. ( a ) Tillering phenotypes. Scale bar, 5 cm. ( b ) miR444a and its target sequence sketch. ( c , d ) Relative expression in the transgenic lines. ( e ) Tiller numbers at 70 DAG. Values represent means±s.e. of ten plants. * P <0.05, ** P <0.01 by Student’s t- test. Full size image OsMADS57 was predicted to be a target of the 21-nt non-coding RNA miR444a ( Fig. 2b ), which is conserved in monocots such as wheat, barley, maize, sorghum and sugarcane [31] . We created OsMIR444a -overexpressing rice lines (miROE; Supplementary Fig. S3 ), and qRT–PCR and RNA gel blot analyses indicated that miR444a transcript levels were increased in these lines compared with WT ( Fig. 2d and Supplementary Fig. S4 ). Correspondingly, OsMADS57 expression was significantly reduced in the miROE lines ( Fig. 2c ). The miROE lines had fewer tillers than did WT, similar to the AS lines ( Fig. 2a ). By contrast, tiller numbers in the miROE lines were altered significantly compared with osmads57-1 ( Fig. 1e ) and OE lines ( Fig. 2a ). The miROE lines were similar to WT ZH10 in root development and floral organogenesis and development ( Supplementary Fig. S2a,c ). These results demonstrate that the expression of OsMADS57 is repressed by OsMIR444a to control tillering. Expression patterns of OsMADS57 and its repressor activity We searched the Genevestigator database, the HANADB-Os database and the eFP browser of rice microarray data [9] , [32] , [33] for OsMADS57 expression data. The results indicated that OsMADS57 expression was higher during tillering and stem-elongation stages than other stages in rice ( Supplementary Fig. S5a ). It was highly expressed in leaf tissues and weakly expressed in other organs ( Supplementary Fig. S5b–d ). Quantitative RT–PCR assays showed that the highest transcript level of OsMADS57 was in sheaths and leaves, and that no signals were observed in the culm ( Fig. 3a ). On the other hand, expression of miR444a was found in all organs except for roots. RNA in situ hybridization assays revealed OsMADS57 expression predominantly in shoot apical meristems and axillary buds ( Fig. 3b ). This suggests that OsMADS57 is involved in the outgrowth of axillary buds. 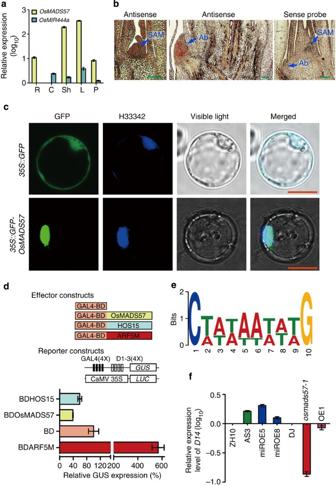Figure 3: Expression patterns ofOsMADS57and its regulation activity. (a) Expression in roots (R), culms (C), sheaths (Sh), leaves (L) and panicles (P). (b) RNAin situhybridization ofOsMADS57in SAM and axillary buds (Ab). Scale bars, 100 μm. (c) Localization of GFP- OsMADS57 in rice protoplasts. H33342, a nuclear staining dye. Scale bars, 10 μm. (d) The transcriptional repression activity assays in Arabidopsis protoplasts. (4X)-D1–3(4X), four upstream GAL4 DNA-binding sites in the promoter ofGUS; CaMV 35S, a promoter ofLUCreporter (the internal control). HOS15, a transcription suppressor, and ARF5M, an activator, were used as the controls. (e) The preferred CArG-box binding motif for OsMADS57 from the expression level and frequency of the 97 regulated genes. (f)D14expression in various lines. Figure 3: Expression patterns of OsMADS57 and its regulation activity. ( a ) Expression in roots (R), culms (C), sheaths (Sh), leaves (L) and panicles (P). ( b ) RNA in situ hybridization of OsMADS57 in SAM and axillary buds (Ab). Scale bars, 100 μm. ( c ) Localization of GFP- OsMADS57 in rice protoplasts. H33342, a nuclear staining dye. Scale bars, 10 μm. ( d ) The transcriptional repression activity assays in Arabidopsis protoplasts. (4X)-D1–3(4X), four upstream GAL4 DNA-binding sites in the promoter of GUS ; CaMV 35S, a promoter of LUC reporter (the internal control). HOS15, a transcription suppressor, and ARF5M, an activator, were used as the controls. ( e ) The preferred CArG-box binding motif for OsMADS57 from the expression level and frequency of the 97 regulated genes. ( f ) D14 expression in various lines. Full size image In subcellular localization assays, green fluorescent protein (GFP)-OsMADS57 fluorescence completely overlapped with H33342 nuclear staining in rice protoplasts ( Fig. 3c ). By contrast, GFP fluorescence of the transgenic control cells was localized in the plasma membrane and cytoplasm. To identify the physical interaction between the regulatory transcription factor OsMADS57 and its DNA targets, a yeast one-hybrid system was used ( Fig. 3d ). Transcriptional activity assays using protoplasts revealed that OsMADS57 fused to the DNA-binding domain from GAL4 (BD), and significantly repressed the expression (40%) of the target reporter gene GUS , which contained four GAL4 DNA-binding sites in the promoter, compared with BD alone (set to 100%). Meanwhile, for the previously reported repressed gene HOS15 (ref. 34 ), which was used as a positive control for the repressor activity, GUS expression was 60% of that with BD alone. The negative control, ARF5M, activated GUS expression 5.8-fold compared with BD only. Therefore, OsMADS57 has the ability to repress transcription of its target genes. Genome-wide gene expression analysis of OsMADS57 To investigate potential target genes of OsMADS57 , we performed Affymetrix rice microarray assays using probes from osmads57-1 and WT DJ ( Supplementary Figs S6 and S7a ). The signal value (log 2 ratio) of OsMADS57 was 2.99 in osmads57-1 , which was similar to our qRT–PCR results ( Fig. 1d and Supplementary Table S1 ). Microarray data analysis revealed that 175 genes upregulated and 19 genes downregulated by more than twofold (|log 2 ratio|≥1) in the osmads57-1 mutant compared with DJ ( Supplementary Fig. S7b and Table S1 ). GO analysis showed that transcription factor-, hormone-, cell division-, metabolism- and membrane-related genes were clustered in up- and downregulated groups ( Supplementary Table S2 ). Genes that have been demonstrated to promote tillering, such as GA2ox4 , GA2ox6 and GA2ox9 , were found among the upregulated genes in the microarray data ( Table 1 ) [18] , [35] , [36] , [37] , [38] . Table 1 Genes of known function in tillering with altered expression patterns in the osmads57-1 mutant based on the microarray data. Full size table MADS-box transcription factors bind to the cis -element CArG box C(T/A)(T/A) (T/A)(T/A)(T/A)(T/A)(T/A)(T/A)G (refs 4 , 6 , 7 , 39 ). We performed cis -element screening in the region −1,500 to −1 bp from the initiation code for all 175 up- and 19 downregulated genes. Among all of the differentially regulated genes, which should include both direct and indirect targets, the CArG cis -element was identified in 86 upregulated genes and 11 downregulated genes ( Supplementary Fig. S7b and Table S3 ). On the basis of MEME suite analysis of the expression level and frequency of the 97 regulated genes, we characterized the preferred CArG box of OsMADS57 ( Fig. 3e ). C 1 xxxxxxxxG 10 was the strongest element contributing to the binding; other important contributors were the elements at (A/T) 5 and (A/T) 6 , as well as (T/A) 2 ( Fig. 3e ). Importantly, the frequencies of the preferred CArG cis -element in random gene sequences from the whole genome were much lower than in the regulated genes ( Supplementary Fig. S7c ). Using the potential OsMADS57-binding motif to search for further target sequences, one of the preferred CArG-box motifs [C(A/T)TTAAAAAG] was found in the promoter of D14 (Os03g10620), which was previously identified as controlling tiller development [20] , [24] , [40] . In our Affymetrix GeneChip assay, unexpectedly, D14 was not among the regulated genes, possibly because of biased probes for D14 on the chip ( Supplementary Fig. S8 and Table S3 ). We examined the expression of D14 by qRT–PCR in lines with various levels of OsMADS57 expression ( Fig. 3f ). D14 transcription was dramatically downregulated in the osmads57-1 mutant, and somewhat downregulated in the OsMADS57 OE line. Conversely, D14 expression was upregulated in the OsMADS57 AS and miROE lines. This suggests that expression of D14 is negatively regulated by OsMADS57 in rice. D14 is a direct target of OsMADS57 Two likely OsMADS57-binding CArG-boxes sites, site 1 [CTTTAAAAAG] and site 2 [CATTAAAAAG], were found at −2,281 to −2,272 bp and −1,320 to −1,311 bp from the initiation of D14 , respectively ( Fig. 4a ) [20] . Electrophoretic mobility shift assays (EMSAs) revealed that the labelled target of either site 1 or 2 bound to OsMADS57-GST was shifted to bigger in the molecular weight on the gel (lanes 4 and 6) as compared with the target alone (lanes 2 and 8), or the negative control (lanes 3 and 9; Fig. 4b ). Additionally, addition of GST antiserum to the binding reactions resulted in two additional retarded bands with increased molecular weight at the top of the lanes (lanes 5 and 7; Fig. 4b ). At the same time, there was a loss of one band in the small-molecular weight on lanes 4–7, respectively, compared the controls. A ChIP assay using OsMADS57 antibody showed that the regions ‘I’ and ‘II’ of the D14 promoter, which included site 1 and site 2 CArG motifs, respectively, were enriched in osmads57-1 compared with WT ( Fig. 4c and Supplementary Fig. S9 ). By contrast, there were no differences for regions ‘III’ and ‘IV’ between osmads57-1 and WT. Thus, OsMADS57 targeted both the CArG cis -elements, site 1 and site 2, that were present in D14 . 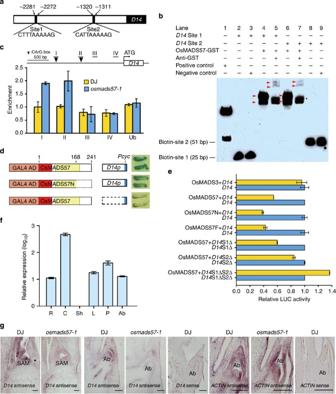Figure 4: OsMADS57 inhibitsD14expression. (a)D14promoter sketch showing CArG-boxes. (b) EMSA of OsMADS57 binding thecis-elements. The amount of protein loaded in each lane was equal. (c) ChIP assay of 2-week-seedling to show OsMADS57-binding regions inD14promoter. Regions I and II contain the probes used in EMSA. TheUBIQUITIN(Ub) promoter was used as a control. (d) Yeast one-hybrid analysis. The effectors contained the GAL4-activation domain. (e) Transcriptional repression activity assay in Arabidopsis protoplasts. S1Δ and/or S2Δ, deletion of site 1 and/or 2. (f)D14expression in roots (R), culms (C), sheaths (Sh), leaves (L), panicles (P) and axillary buds(Ab). (g) RNAin situassay forD14. Scale bars, 100 μm. Figure 4: OsMADS57 inhibits D14 expression. ( a ) D14 promoter sketch showing CArG-boxes. ( b ) EMSA of OsMADS57 binding the cis -elements. The amount of protein loaded in each lane was equal. ( c ) ChIP assay of 2-week-seedling to show OsMADS57-binding regions in D14 promoter. Regions I and II contain the probes used in EMSA. The UBIQUITIN (Ub) promoter was used as a control. ( d ) Yeast one-hybrid analysis. The effectors contained the GAL4-activation domain. ( e ) Transcriptional repression activity assay in Arabidopsis protoplasts. S1Δ and/or S2Δ, deletion of site 1 and/or 2. ( f ) D14 expression in roots (R), culms (C), sheaths (Sh), leaves (L), panicles (P) and axillary buds(Ab). ( g ) RNA in situ assay for D14 . Scale bars, 100 μm. Full size image The activities of OsMADS57 and an N-terminal peptide of 168 amino-acid residues (OsMADS57N) were analysed in yeast via expression of the reporter gene LacZ driven by the D14 promoter- Pcyc1 ( D14p ). The effectors contained the GAL4-activation domain. The strains with the full-length or truncated genes grew well and were blue compared with the control ( Fig. 4d ). By contrast, yeast cells with OsMADS57 , but lacking the D14 promoter, did not turn blue. Therefore, the truncated protein bound to the D14 promoter in yeast, as did the full-length gene. A transcriptional regulation activity assay in protoplasts revealed that OsMADS57, OsMADS57N and the fusion protein OsMADS57F repressed the expression of the D14 promoter driving the luciferase ( LUC ) reporter gene ( Fig. 4e ). On the other hand, the inhibition of OsMADS57 on D14 was diminished by deleting the site 2 CArG box. When both binding sites were deleted from D14 , OsMADS57 showed a increased LUC expression in the assay system ( Fig. 4e ). Therefore, OsMADS57 requires those sites to repress D14 transcription. Quantitative RT–PCR analyses revealed that D14 expression was high in culms, but low in roots, leaves, panicles and axillary buds ( Fig. 4f ). RNA in situ hybridization demonstrated that D14 transcripts were prominent at the shoot apical meristem (SAM) and axillary buds in WT, but were reduced in osmads57-1 tissues ( Fig. 4g ). By contrast, in situ expression analysis of the ACTIN gene as a control showed no obvious difference between osmads57-1 and WT. The expression pattern of D14 overlapped with that of OsMADS57 in the SAM and axillary buds ( Fig. 3b ). qRT–PCR assays revealed that the D14 mRNA level was suppressed in osmads57-1 in planta ( Fig. 3f ). Therefore, OsMADS57 seems to target D14 directly to suppress its transcription in rice. A loss-of-function d14 mutant had a dwarf phenotype and a huge number of tillers (46 tillers per plant), whereas the gain-of-function osmads57-1 mutant had a weak dwarf phenotype and a somewhat increased number of tillers (28 tillers per plant) ( Fig. 5a and Supplementary Table S4 ). d14osmads57-1 -double mutant plants (including both D14 −/− OsMADS57 −/− and D14 −/− OsMADS + /− ) had a clearly elevated number of tillers (55 tillers per plant) and a dwarf phenotype, similar to the parental d14 line, but dissimilar from the osmads57-1 parent. d14 is in a Shoikari (Shi) background, while osmads57-1 is in the DJ background. WT plants of these backgrounds did not differ significantly in the tillering phenotype. As such, genetic analysis demonstrates that OsMADS57 is functionally dependent on D14 . 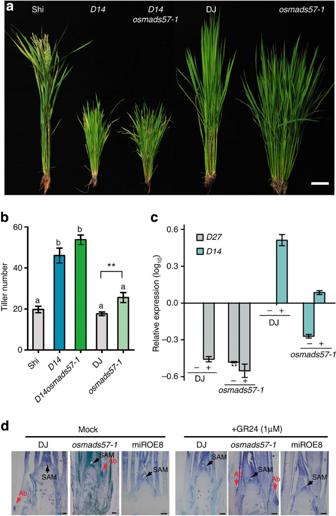Figure 5: Double mutantd14osmads57-1and response to GR24. (a,b) Tiller phenotypes and tiller number at heading stage. Scale bar, 10 cm. Different letters a and b represent significant differences among the lines (the least significant difference test,P<0.05). **P<0.01 by Student’st-test. (c)D27andD14expression with (+) or without (−) 1 μM GR24. (d) Longitudinal sections of shoot apex treated with 1 μM GR24. Scale bars, 100 μm. Figure 5: Double mutant d14osmads57-1 and response to GR24. ( a , b ) Tiller phenotypes and tiller number at heading stage. Scale bar, 10 cm. Different letters a and b represent significant differences among the lines (the least significant difference test, P <0.05). ** P <0.01 by Student’s t- test. ( c ) D27 and D14 expression with (+) or without (−) 1 μM GR24. ( d ) Longitudinal sections of shoot apex treated with 1 μM GR24. Scale bars, 100 μm. Full size image To explore the physiological correlation between SL signals and OsMADS57 , the effects of SL on the transcription of D14 (SL signalling) and D27 (SL biosynthesis) were monitored in the osmads57-1 . The expression level of untreated WT (DJ) was defined as the benchmark in qRT–PCR ( Fig. 5c ). The treatment of a synthetic SL, GR24, resulted in a decrease of D27 transcription in both DJ and osmads57-1 . This decrease was much more pronounced in osmads57-1 than in DJ. Untreated osmads57-1 showed a dramatically lower transcriptional level of D27 compared with DJ, which may mimic the effect of GR24 on DJ. D14 expression was induced by GR24 treatment in DJ and osmads57-1 . In the non-treatment condition, the expression level of D14 was obviously lower in osmads57-1 than in DJ. Phenotypically, the outgrowth of axillary buds was repressed by GR24 treatment in DJ ( Fig. 5d ). In contrast, the repression was abolished in osmads57-1 , which was similar to the SL-insensitive phenotype of the d14 mutant [20] , [24] . Regardless of the treatment, the miROE line showed no axillary buds at the same developmental stage. They suggest that OsMADS57 may be involved in SL signalling through D14 in tillering of rice. Transcription activity of OsMADS57 was affected by OsTB1 The rice mutant tb1/fc1 has increased tillering, which is similar to osmads57-1 ( Fig. 1e–g ) and d14 (refs 12 , 15 . Yeast two-hybrid (Y2H) assays showed that yeast cells cotransformed with constructs lacking its C-terminal region (OsMADS57N) could support growth in the selection medium and β-galactosidase staining ( Fig. 6a ). Thus, the truncated OsMADS57 lacking its intact C-terminal region (OsMADS57N) was sufficient to interact with OsMADS57. Y2H assays indicated that the interaction between OsTB1 and OsMADS57 appeared in yeast cells, and that OsTB1 was self-activated ( Fig. 6b ). Therefore, OsMADS57 was able to form a heterodimer with OsTB1. 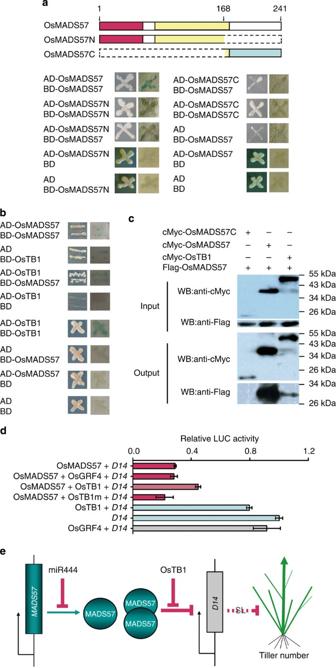Figure 6: OsMADS57 interaction with OsTB1. (a,b) Yeast two-hybrid assay. Diagrams represent the proteins. Yeast strains were grown on synthetic dropout medium lacking Trp, Leu, His and Ade, and stained for β-galactosidase activity. (c) Co-IP assay in Arabidopsis protoplasts. OsMADS57C, C-terminal 169–241 amino acids. (d) Effect of OsTB1 and OsTB1A159QWA162A163(OsTB1m) on transcriptional regulation ofD14via OsMADS57 in protoplasts. (e) Model of the OsMADS57-mediated network for control of tillering. WB, western blot. Figure 6: OsMADS57 interaction with OsTB1. ( a , b ) Yeast two-hybrid assay. Diagrams represent the proteins. Yeast strains were grown on synthetic dropout medium lacking Trp, Leu, His and Ade, and stained for β-galactosidase activity. ( c ) Co-IP assay in Arabidopsis protoplasts. OsMADS57C, C-terminal 169–241 amino acids. ( d ) Effect of OsTB1 and OsTB1 A 159QW A 162 A 163 (OsTB1m) on transcriptional regulation of D14 via OsMADS57 in protoplasts. ( e ) Model of the OsMADS57-mediated network for control of tillering. WB, western blot. Full size image Co-immunoprecipitation (Co-IP) tests revealed that the protein complexes pulled down by anti-c-Myc agarose were recognized by anti-Flag antibody in lines cotransformed with cMyc-OsMADS57 and Flag-OsMADS57 , or with cMyc-OsTB1 and Flag-OsMADS57 ( Fig. 6c ). Therefore, OsMADS57 could bind to itself and/or to OsTB1 in planta . Expression of D14::LUC was significantly repressed by OsMADS57 in protoplasts ( Fig. 6d ). By contrast, the extent of D14::LUC repression was reduced by cotransformation with OsTB1 . When OsMADS57 and a mutated version OsTB1 A 159QW A 162 A 163 were cotransformed, the activity pattern of D14::LUC was the same as OsMADS57 alone. OsTB1 alone did not obviously disturb the activity of D14::LUC in the system. A negative control, OsGRF4, did not affect D14::LUC activity ( Fig. 6d ). Therefore, OsMADS57 interacted directly with OsTB1, and this interaction could partially relieve the inhibitory effect of OsMADS57 on D14 transcription ( Fig. 6e ). miR444a-dependent OsMADS57 regulates tiller development In the model of MADS-box gene-mediated regulation of floral organogenesis and flowering, MADS transcription factors exert their function by forming homodimers or heterodimers, recognizing and binding the cis -element CArG boxes, and then regulating the expression of target genes [6] , [8] , [41] . The M-, I- and K-domains in MADS-box homeotic proteins lacking the C-terminal domain are sufficient for several MADS-box proteins to exert their functions in the investigated examples [4] , [42] , [43] . In the AGL2 -like clade, the truncated proteins AGL1 and AGL2 lack the C-terminal domain, but can form homodimers and heterodimers and bind to the CArG boxes in vitro [4] , [42] , [43] . In this study, we demonstrated that the truncated OsMADS57 protein lacking an intact C-terminus was able to form dimers. The truncated OsMADS57 gene acted as a gain-of-function gene for tiller development in the activation-tagged mutant osmads57-1 . OsMADS57 also directly interacted with the TCP transcription factor OsTB1 at the protein level ( Fig. 6 ). OsTB1 interaction with OsMADS57 reduced the negative regulation activity of OsMADS57 on D14 expression, through which OsMADS57 affected tillering ( Fig. 5a ). The OsMADS57 and OsTB1 genes were expressed together at the shoot apical meristem and axillary buds. Our gain-of-function mutant osmads57-1 and the loss-of-function mutant ostb1/fc1 both had increased tillers, consistent with them acting in the same genetic pathway in rice ( Figs 1 and 5 ) [12] , [15] . OsTB1 is a negative regulator controlling tiller outgrowth, whereas OsMADS57 is a positive regulator. Therefore, our data support the hypothesis that OsMADS57 can interact with OsTB1 to mediate transcriptional regulation of target genes, such as D14 , and impact the outgrowth of axillary buds ( Fig. 6e ). This serves as another example of MADS and TCP family members directly functioning in vegetative organogenesis and development, as has been demonstrated for floral organogenesis in Arabidopsis [12] , [13] , [14] . Our data on the expression patterns of miR444a and OsMADS57 , as well as the phenotypic analysis of the transgenic lines, support the prediction that miR444a directly targets OsMADS57 to knockdown its transcript level and regulate tillering in rice ( Fig. 2 ) [31] , [44] . Phenotypically, overexpression of miR444a resulted in decreased transcript levels of the OsMADS57 gene and reduced tillering. As would be expected, this phenotype was similar to that of the OsMADS57 antisense lines, but significantly different from that of the OsMADS57 -overexpression lines, which showed increased tiller numbers ( Fig. 2 ). As downregulation of OsMADS57 expression mediated by miR444a suppressed tillering, it can be concluded that miR444a-dependent OsMADS57 is involved in the regulation of tillering during rice development ( Fig. 6e ). OsMADS57 directly repressed D14 transcription to regulate tiller organogenesis SL signalling and biosynthesis are involved in the regulation of branching in plants. DAD2, an orthologue of D14 in petunia, functions in SL perception and signalling. DAD2 binds to SL and interacts with the F-box protein PhMAX2A. The hydrolysis or binding of SL by DAD2 is required for DAD2 destabilization by the SCF (SKP1-CULLIN1-F-box) complex, which mediates signalling to regulate tillering [25] . D27 and D14 genes genetically function in the MAX / RMS / D pathway of SL biosynthesis [15] , [17] , [18] , [26] , [27] . It is possible that the function of D14 in biosynthesis is likely a feedback effect of SL signalling. Analysis of the d14osmads57-1 -double mutant indicated that OsMADS57 was functionally dependent on D14/D88 in rice tillering ( Fig. 5 ). The osmads57-1 mutant was insensitive to SL, similar to d14 . The negative effect of SL on D27 expression, as well as the abolished SL inhibition of outgrowth in osmads57-1 , suggest that OsMADS57 is involved in D14 function in the SL pathway to regulate tillering. OsMADS57 interacted with OsTB1 and regulated tiller development in rice ( Fig. 6 ). OsTB1/FC1 functions in the SL pathway to inhibit outgrowth of axillary buds, and is an integrator of multiple signalling pathways in rice [15] , [45] . The spatial expression pattern of OsMADS57 is similar to OsTB1/FC1 in axillary buds ( Fig. 4 ) [15] , [45] , and OsMADS57 physically interacted with OsTB1/FC1 ( Fig. 6 ). OsMADS57 may be involved in balancing the D14 -mediated SL signalling pathway through its protein interaction with OsTB1/FC1 (ref. 15 ). The gain-of-function mutants osmads57-1 and ostb1/fc1 , as well as the loss-of-function mutant d14 were insensitive to SL treatment ( Fig. 5 ) [20] , [21] , [24] , [40] . At the protein level, OsMADS57 physically interacted with OsTB1/FC1 to regulate D14 expression, and requires the V 159 XXL 162 L 163 motif in OsTB1 ( Fig.6 ) [15] , [46] . The VXXLL motif is a signature sequence in the transcriptional coactivators and mediates binding to liganded nuclear receptors in animal cells [47] . Consistently, OsTB1/FC1 functions as a negative regulator of the SL signalling pathway [15] . It is possible that OsMADS57 is required for the SL signalling pathway to inhibit bud growth. D14 expression was downregulated in the osmads57-1 mutant. The SL-mediated induction of D14 expression remains strong in osmads57-1 (>2-fold), although it was less than that in WT. This suggests that SL-induced D14 expression is counterbalanced by the repression of OsMADS57 on transcription. Together, our data indicate that OsMADS57, along with OsTB1, regulates the expression of D14 ( Fig. 6e ). MADS-box transcription factors recognize cis -element CArG boxes. Our data from the binding and transcription assays suggest that OsMADS57 interacts with its preferred CArG-box motif [C(A/T)TTAAAAAG] in the promoter of the D14 gene to suppress expression. The transcriptional repression activity of OsMADS57 on D14 was reduced by its protein interaction with OsTB1 as a heterodimer ( Fig. 6 ). In the transgenic lines, as well as the osmads57-1 mutant, D14 expression was negatively regulated by OsMADS57 in planta ( Fig. 4g ). Thus, the MADS and TCP complexes with homodimer and/or heterodimer may be involved in regulating branching [48] . Opposite tillering phenotypes were observed between the loss-of-function ostb1 and the OsMADS57 -knockdown lines of overexpressing miR444a or antisense OsMADS57 , whereas similar phenotypes were found in ostb1 and the gain-of-function osmads57-1. D14 expression was reduced at the axillary buds in osmads57-1 ( Figs 3f and 4g ), which is consistent with the phenotype of the d14 mutant [20] , [24] . Together, this suggests that the interactions of MADS-box (OsMADS57) and TCP (OsTB1) transcription factors result in a dynamic balance of the target gene expression during tillering. This finding enhances our understanding of the function of this conserved MADS-box protein and its mediating network involving well-known genes, such as OsTB1 and D14 , that are known to control tillering [15] , [20] . In summary, tillering in rice involves a miRNA/MADS/TCP/D14 (miMTD) regulation module or network, in which OsMADS57, modulated by its interaction with OsTB1, directly represses D14 expression, which is in turn involved in SL perception and signalling [25] . Furthermore, the OsMADS57 gene is targeted and regulated negatively by miR444a. The discovery of such a miMTD regulation mechanism for tillering has great potential application for use in efforts to increase yields through rice molecular breeding programs. Plant materials The T-DNA insertion mutant line PFG_3A-05432.L ( osmads57-1 ) in an Oryza sativa ssp japonica cv Dongjin background was obtained from RiceGE, the Rice Functional Genomics Express Database, in Pohang city, Korea. The d14/d88 mutant was a gift from Qian’s lab, China Insititute of Rice Biology. All transgenic lines were developed in the genetic background of O. sativa ssp japonica cv Zhonghua10 (ZH10). Rice plants were grown in a temperature-controlled greenhouse with 30 °C/25 °C day/night cycles. The analysis of tiller numbers used materials from ten plants from each line. Developing axillary buds from osmads57-1 and Dongjin 30 DAG were used in the microarray experiments. Transformation of rice plants Genetic transformation of rice plants was performed using Agrobacterium -mediated methods. Full-length cDNA of the OsMADS57 gene in a sense orientation was used for the overexpression construct. The OsMADS57 gene in an antisense orientation was used for the antisense construct. The constructed vectors were transformed with the use of Agrobacterium tumefaciens strain EHA105. All primers used in the study are presented in Supplementary Table S5 . Quantitative RT–PCR Total RNA was extracted using a TRIzol RNA extraction kit (Invitrogen) and treated with RNase-free DNase I (MBI Fermentas). RNA was used to synthesize cDNA using AMV Reverse Transcriptase (Promega). Quantitative RT–PCR was performed on a Mx3000P instrument (Stratagene) with SYBR Green Real-time PCR Master Mix (Toyobo) according to the manufacturer’s instructions. Gene expression was normalized to that of ACTIN. miRNA levels were normalized to 5.8S rRNA levels by qRT–PCR. The relative expression level (log 10 ) in the WT ZH10 line was defined as 0. Experiments included three technical replicates and at least three biological replicates. Values represent means±s.e. of three technical replicates. Primers used for qRT–PCR are presented in Supplementary Table S5 . In situ hybridization In situ hybridization was performed as described previously [49] . Digoxigenin-labelled hybrid probes were transcribed in vitro from cDNA of OsMADS57 , ACTIN and D14 with gene-specific primers ( Supplementary Table S5 ). SAM and axillary buds were used for hybridization assays. Slides were photographed under a microscope (Zeiss). Yeast one-hybrid assays Yeast one-hybrid assays were used to check binding of OsMADS57 to D14 [50] . cDNA encoding full-length OsMADS57 and OsMADS57N (amino acids 1–168) were inserted into pGAD424 to generate pGAD424-OsMADS57 and pGAD424-OsMADS57N, respectively. The effectors contained the GAL4-activation domain. To generate the D14p-Pcyc1::LacZ reporter plasmid, a D14 promoter was amplified with the primers D14pEcoRIF and D14XhoIR. These constructs were transformed into the Saccharomyces cerevisiae strain EGY48. Transformed yeast was selected on synthetic complete medium lacking Ura and Leu [50] . Yeast two-hybrid assays The cDNAs for OsMADS57, OsMADS57N, OsMADS57C, OsTB1 and OsTB1 A 159QW A 162 A 163 were cloned into the pGADT7 and pGBKT7 (Stratagene) vectors. These constructs were transformed into S. cerevisiae strain AH109. Individual colonies of transformants were screened by growing on medium lacking Leu, Trp and His. Recovered clones were transferred onto a filter paper and then assayed for LacZ activity. Protoplast transformation and transient expression assays The transcription activity assay was carried out in the transient-transformed protoplast. The DNA-binding domain (BD) from GAL4 was used in the system [34] . The GAL4 BD–OsMADS57 fusion protein can bind to the GAL4 DNA-binding sites of the GUS reporter. Two known proteins HOS15, a transcription suppressor, and ARF5M, an activator, were used as the controls. The GUS reporter containing four upstream GAL4 DNA-binding sites ( GAL4 (4X)-D1-3(4X)- GUS ) and the luciferase ( LUC ) reporter were cotransformed with GAL4 BD–OsMADS57 into Arabidopsis protoplasts. The LUC reporter carrying the luciferase gene under control of CaMV 35S promoter was used as the internal control to normalize the data for eliminating variations in the experiment. For the specific binding and repressing activity to D14 promoter assay, OsMADS57 and its mutated forms were used in the system [50] . The cDNAs for full-length OsMADS57 , OsMADS57N , and OsMADS57F were fused into the pBI221 vector driven by the 35S promoter to generate pBI221-OsMADS57, pBI221-OsMADS57N and pBI221-OsMADS57F, respectively. To generate the D14:LUC reporter gene, the D14 promoter was amplified. The plasmid carrying the GUS gene under the control of the 35S promoter was used as a normalization control. Values represent means±s.e. of three technical replicates. Cotransformation of OsMADS57 and OsTB1 was done for identifying effect of OsTB1 in the transient assay. As a control, OsTB1 V 159QW L 162 L 163 was replaced with OsTB1 A 159QW A 162 A 163 to disturb its interaction with OsMADS57 (ref. 47 ). Electrophoretic mobility shift assays EMSAs were performed to identify the binding activity of OsMADS57 to the potential motifs [51] . Oligonucleotides complementary to different motifs of the D14 promoter were synthesized and labelled using a Biotin 3′ End DNA Labeling Kit (Pierce). For supershift assays, anti-GST antiserum (Sigma-Aldrich) was added to the reaction. Chromatin immunoprecipitation assays To confirm the binding activity of OsMADS57 to D14 in vivo , chromatin immunoprecipitation (ChIP) assay was carried out using the root-dislodged 2-week-old seedlings [52] . Purified anti-OsMADS57 polyclonal antibody (BGI, Beijing) was used for IP. As negative controls, an agarose/Salmon sperm DNA (Millipore) with the preimmune serum was used. The DNA products of IP were analysed by qRT–PCR. The enrichment was calculated as the ratio of osmads57-1 to DJ (I). Data are mean±s.d. of three independent experiments. The primers used in the ChIP assays are listed in Supplementary Table S5 . Co-IP assays To validate the proteins interaction of OsMADS57 and OsTB1 in vivo , Co-IP assay approach was used [53] . The cDNAs for OsMADS57 , OsMADS57C and OsTB1 were amplified using the primers MSNCFBamHI and MSNCRKpnI, OsMADS57BamHIF and OsMADS57KpnIR, and OsTB1BamHI sense and OsTB1KpnI antisense, respectively. Amplified cDNAs were inserted into pRT107-6XMyc or pRT105-3XFlag [53] between BamHI and KpnI sites to generate the four expression vectors 2 × 35S::6XMyc-OsMADS57C , 2 × 35S::6XMyc-OsMADS57 , 2 × 35S::3XFag-OsMADS57 and 2 × 35S::6XMyc-OsTB1. Protoplasts from Arabidopsis thaliana (Col-0) were isolated and transformed using a polyethylene glycol-mediated technique [54] . Both anti-c-Myc and anti-Flag antibodies (Sigma-Aldrich) were used. The crude protein extract was used as input and the products pulled down by the anti-c-Myc agarose conjugate were used as output. All primers used in the study are presented in Supplementary Table S5 . Histological analyses Seedlings were treated with 1 μM GR24 in Kimura B nutrient solution [55] for 8 days. Tissues of SAM and axillary buds from 15-day-old plants were fixed and sectioned into 7-μm sections and stained with toluidine blue or fuschin red for light microscopic analysis (Zeiss). Subcellular localization of fusion protein in protoplast A transient expression vector, 35S:GFP-OsMADS57, was constructed. For protoplast transformation, the released protoplast cells from leaf sheaths of 10-day-old etiolated rice seedlings were isolated and transformed via the polyethylene glycol (PEG 4000) method [56] . At the same time, Hoechst 33342 was used to stain the nucleic acids that were then visualized at an excitation wavelength of 405 nm. Phylogenetic analysis The phylogenetic analysis of 20 MADS-box protein sequences from Arabidopsis, rice, maize and wheat was performed using MEGA 4.0, with default settings and the neighbour-joining method. Bootstrap values (%) of 2,000 replicates are shown at the branching points. How to cite this article: Guo, S. et al. The interaction between OsMADS57 and OsTB1 modulates rice tillering via DWARF14 . Nat. Commun. 4:1566 doi: 10.1038/ncomms2542 (2013).